Theory of low-power ultra-broadband terahertz sideband generation in bi-layer graphene In a semiconductor illuminated by a strong terahertz (THz) field, optically excited electron–hole pairs can recombine to emit light in a broad frequency comb evenly spaced by twice the THz frequency. Such high-order THz sideband generation is of interest both as an example of extreme nonlinear optics and also as a method for ultrafast electro-optical modulation. So far, this phenomenon has only been observed with large field strengths (~10 kV cm −1 ), an obstacle for technological applications. Here we predict that bi-layer graphene generates high-order sidebands at much weaker THz fields. We find that a THz field of strength 1 kV cm −1 can produce a high-sideband spectrum of about 30 THz, 100 times broader than in GaAs. The sidebands are generated despite the absence of classical collisions, with the quantum coherence of the electron–hole pairs enabling recombination. These remarkable features lower the barrier to desktop electro-optical modulation at THz frequencies, facilitating ultrafast optical communications. The optical modulation that occurs when an intense light field interacts with matter has a wide range of applications, from molecular imaging [1] , [2] to soft X-ray generation [3] , [4] , [5] and potential applications in all-optical signal processing. The well-known process of high-harmonic generation (HHG) [6] —where the interaction of an optical field with an atom results in the emission light in a broad frequency comb evenly spaced by twice the optical field frequency—is an example of such a process. HHG can be understood with a three-step model. In the first step, an electron is ionized from an atom by an intense field. In the second, the ionized electron is accelerated by the field along a closed orbit, returning to the ion at a later time with a higher energy. Finally, the electron recombines with the ion releasing a photon, which is an odd harmonic of the original field. One important feature of the process is its ‘non-perturbative’ nature, which results in a ‘plateau-like’ spectrum where the intensity of the harmonics remains approximately constant up to a cutoff frequency of I p +3.17 U p (where I p is the atom-binding energy and is the ponderomotive energy with E and ω the strength and angular frequency of the light field and e and m e the charge and mass of the driven electron, respectively), outside of which the harmonic strength decays away exponentially [7] , [8] , [9] . The similar process of high-order sideband generation (HSG) can occur in semiconductors [10] . In HSG, a weak optical field promotes a valence band electron to the conduction band, creating an electron–hole pair. The pair is then driven in the band by an intense, terahertz (THz) frequency field. In analogy with HHG, the recombination of the electron–hole pair also produces light in a broad frequency comb ( Fig. 1a ). However, in this case, the resulting sidebands in the excitation field spectrum occur at even harmonics of the THz field. As with HHG, a ‘non-perturbative’ plateau occurs with a cutoff of Δ+3.17 U p (where Δ is the detuning of laser from the band gap of the semiconductor and is the ponderomotive energy with E THz and ω THz , the strength and angular frequency of the THz field and m R the electron-hole reduced mass). Such high-order THz sideband generation is not only of fundamental interest, as an example of extreme nonlinear optics in condensed matter systems, but also of technological importance as a mechanism for ultrafast electro-optical modulation—a crucial ingredient in Tbit s −1 rate optical communication. Hence, HSG has a wide range of potential applications but there is a serious technological challenge; HSG requires large THz field strengths. Current experimental observations of HSG have employed THz field amplitudes on the order of 10 kV cm −1 (ref. 11 ) generated by a free-electron laser [12] , [13] . The need for such large field strengths presents an obstacle to the use of HSG in optical devices. 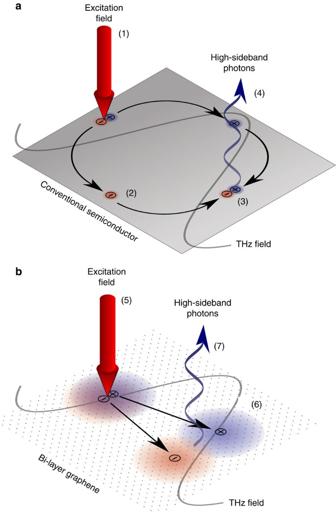Figure 1: Schematics of high-sideband generation in conventional semiconductors and in graphene. (a) In a conventional semiconductor, an electron–hole pair, created by a weak excitation field (1), is accelerated by an intense THz frequency field gaining energy. The electron and hole wavefunctions separate completely (2). The THz field drives the electron and hole back towards each other, recombining (3) and releasing a high-sideband photon (4). (b) In graphene, a weak excitation field excites an electron–hole pair (5), which is accelerated in opposite directions by the THz field (6). As the electron–hole pair has vanishing effective mass, the THz alters their energy and momentum but not their velocity. Hence, the electron and hole separate at the Fermi velocity. However, owing to the broad wavefunction of the electron and hole, there is still significant overlap at finite separations and, hence, recombination (and the release of a high-sideband photon) is possible even though the classical locations of the electron and hole do not coincide (7). Figure 1: Schematics of high-sideband generation in conventional semiconductors and in graphene. ( a ) In a conventional semiconductor, an electron–hole pair, created by a weak excitation field (1), is accelerated by an intense THz frequency field gaining energy. The electron and hole wavefunctions separate completely (2). The THz field drives the electron and hole back towards each other, recombining (3) and releasing a high-sideband photon (4). ( b ) In graphene, a weak excitation field excites an electron–hole pair (5), which is accelerated in opposite directions by the THz field (6). As the electron–hole pair has vanishing effective mass, the THz alters their energy and momentum but not their velocity. Hence, the electron and hole separate at the Fermi velocity. However, owing to the broad wavefunction of the electron and hole, there is still significant overlap at finite separations and, hence, recombination (and the release of a high-sideband photon) is possible even though the classical locations of the electron and hole do not coincide (7). Full size image Novel materials, such as graphene, offer a potential solution to this problem. The maximum modulation bandwidth is given by the maximum kinetic energy that can be obtained from the THz field by the electron–hole pair. This, in turn, is given by the work done on the electron–hole pair by the THz field, ∫ eE THz ν dt , which is linearly proportional to their velocity, ν . Electrons in graphene act like massless Dirac electrons and hence have a large initial velocity ( ν f ≈10 6 ms −1 ). Conversely, electrons in conventional parabolic band semiconductors have vanishing initial velocity near the band edge (although such velocities are available away from the band edge). Hence, graphene’s linear dispersion and ballistic electrons offer a significant energy gain, at least at low energies, over the parabolic bands of traditional semiconductor and, therefore, is a promising candidate material for HSG at the low-field intensities, which would be suitable for optical device design. In addition, graphene’s resonant transition at telecomm frequencies [14] , weak uniform absorptive loss [15] and ultrafast optical response [16] makes it an ideal candidate for optical communication applications. In fact, it has been demonstrated that graphene, owing to its ultrafast electrical response, is a promising material for ultrafast electro-optical modulation [17] . Here we report on the prediction that, although conversion efficiency is much lower, bi-layer graphene (BLG) [18] , [19] , [20] produces a much broader bandwidth of modulation than conventional semiconductors and, specifically, BLG is a versatile system for HSG at telecommunication wavelength (1.55 μm). We find that a THz field of strength 1 kV cm −1 can produce an HSG spectrum of about 30 THz in the telecom waveband, 100 times broader than in GaAs (or, equivalently, a comparable bandwidth in GaAs would require THz field intensities that are 100 times stronger). These remarkable features make it possible to realize HSG with a much weaker THz laser, which lowers the barrier to desktop electro-optical modulation at THz frequencies, facilitating ultrafast optical communication. HSG in the absence of classical collisions The analysis of HSG in a conventional semiconductor is semi-classical; the sideband spectrum is found from the optical emission associated with the classical collision of electron–hole pairs that have been driven along closed trajectories ( Fig. 1a ). From a semi-classical perspective, however, HSG in graphene seems impossible. Optically excited electron–hole pairs, owing to their massless nature, act like photons in that their velocity is fixed at the Fermi velocity. The action of the THz field changes the momentum and energy of the electron and hole, but the velocity remains constant. As a result, the electron and hole separate at a constant rate and do not return to the same location ( Fig. 1b ) and, hence, no classical collisions occur. A similar issue is shared by electron–hole pairs excited well above the band edge. In this regime, the carriers, as with graphene, are created with a large initial velocity but, again, the THz field is usually not strong enough to reverse their direction of motion and classical collisions are absent. Recent work has shown that HSG can still be created in the absence of classical collisions if the coherence time of the electron–hole pairs is longer than half the THz period [21] (also see Supplementary Note 1 and Supplementary Fig. 1 ). The long coherence time leads to broad electron and hole wavefunctions that can overlap significantly, even when the classical separation is non-zero. Hence, the electron and hole can still recombine to form sidebands even in the absence of classical collisions. As the semi-classical collisions are absent in graphene, it is this ‘quantum’ process that is the dominant mechanism of HSG in this material. Furthermore, the absence of the recollision condition means that the carriers can be accelerated by the THz field for the full half cycle and hence attain an energy that is greater than the Δ+3.17 U p limit imposed by the necessity of classical recollision. Thus, this quantum coherence-induced sideband plateau is broader than the semi-classical plateau. HSG in BLG In the following study, the optical spectrum of a THz-driven electron–hole pair in biased BLG is investigated. We consider BLG, as opposed to monolayer graphene, as a bias field can be applied to the dual layer structure to open a gap at the Dirac point [22] ( Fig. 2a ), which avoids excitations of many electron–hole pairs by the THz field (Schwinger instability [23] ), while still maintaining linear dispersion at the telecomm frequencies. The low-energy band structure of BLG [19] , [20] (also see Supplementary Note 2 ) displays four valley-degenerate bands, of which the two of lower energy, E v and E v′ , are fully occupied valence bands and the two of higher energy, E c and E c′ , are fully empty conduction bands ( Fig. 2b ). With a relatively low-intensity THz field and an excitation field in the C-band of the telecomm frequency range only one of the four possible transitions is significant. The major contribution to the spectrum comes from the E v → E c transition (labelled (4) in Fig. 2b ), where both the electron and hole are created in the linear-dispersion region. This is where the initial velocity is highest and hence where the maximum kinetic energy gain can be obtained. The other transitions (labelled (1–3) in Fig. 2b ) contribute to a lesser extent to the HSG spectrum as either the electron or the hole is created in the parabolic-dispersion region or the optical excitation is off resonant or both (the HSG spectrum due to transitions 1 and 3 is narrower by approximately a factor of two and the HSG due to transition 2 is negligible). Thus, the maximum modulation is determined by E v → E c transition alone. 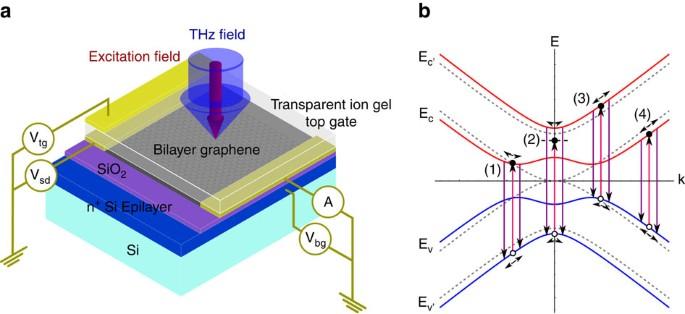Figure 2: Device structure and mechanism for high-sideband generation in bi-layer graphene. (a) Device design for high-sideband generation. A single sheet of BLG is layered on a silicon dioxide substrate and biased via a gate voltage. The top gate is transparent in order to allow the incident THz and optical excitation fields to reach the graphene layer. The n+Si epilayer should be thin compared with the penetration depth of the THz field in order to avoid significant reflection. (b) Acceleration of electrons/holes along the energy bands. The grey dashed curves show the band structure for unbiased BLG. The four hyperbolic bands are gapless at the Dirac point rendering the material a semi-metal. The application of a bias field opens a gap at the Dirac point, converting BLG from a semi-metal to a semi-conductor. The 1.55 μm excitation field creates electron–hole pairs, via three resonant transitions ((1), (3) and (4)) and one off-resonant transition (2). These electron–hole pairs are then driven in the band, recombining to produce the optical sideband spectrum. The dominant contribution is from the transition between theEv→Ec(4), which occurs in the linear region of the bands. Figure 2: Device structure and mechanism for high-sideband generation in bi-layer graphene. ( a ) Device design for high-sideband generation. A single sheet of BLG is layered on a silicon dioxide substrate and biased via a gate voltage. The top gate is transparent in order to allow the incident THz and optical excitation fields to reach the graphene layer. The n + Si epilayer should be thin compared with the penetration depth of the THz field in order to avoid significant reflection. ( b ) Acceleration of electrons/holes along the energy bands. The grey dashed curves show the band structure for unbiased BLG. The four hyperbolic bands are gapless at the Dirac point rendering the material a semi-metal. The application of a bias field opens a gap at the Dirac point, converting BLG from a semi-metal to a semi-conductor. The 1.55 μm excitation field creates electron–hole pairs, via three resonant transitions ((1), (3) and (4)) and one off-resonant transition (2). These electron–hole pairs are then driven in the band, recombining to produce the optical sideband spectrum. The dominant contribution is from the transition between the E v → E c (4), which occurs in the linear region of the bands. Full size image We treat the THz-field as a continuous wave of the form, F THz ( t )= F THz cos( ω THz t ), which we take to be polarized in the x -direction. Similarly, the weak excitation field is taken to be a continuous wave, . The coupling of the THz field to the material is introduced via the time-dependent canonical momentum by the inclusion of the vector potential with . If the excitation field is sufficiently weak, then one can work in the quasi-equilibrium regime, where the depletion of the valence band is negligible. We also note that the large gap induced by the bias field prevents interband transitions caused by the THz field. These facts allow us to work in the single active electron approximation and, hence, ignore electron–electron correlation effects. Simulation parameters and results We evaluate this system by direct simulation of the time-dependent Schrödinger equation for an excitation field of 1.55 μm (194 THz), which is located in the C-band of the telecomm frequencies, and a THz field of frequency 1 THz. The energy gap induced by the bias voltage on the BLG was set to 0.28 eV, which is achievable with a field of ~3 V nm −1 (ref. 22 ). The dephasing factor, Γ, is introduced to account for various relaxation mechanisms. Studies of hot carrier relaxation in monolayer graphene and BLG have shown that carrier lifetimes are on the order of 100 s of femtoseconds [24] , [25] , [26] . However, these studies have been performed at high pump intensities (for example, ~6 × 10 5 mW μm −2 (ref. 24 ). At such high intensities, one expects dense carrier concentrations on the order of 10 13 cm −2 . In this regime, fast carrier–carrier scattering will dominate. HSG experiments are conducted at much lower pump intensities (~3 × 10 −4 mW μm −2 ) (ref. 11 ) and the resulting low carrier concentrations will lead to a suppression of the carrier–carrier scattering rate. Simulations that include both carrier–carrier and carrier–phonon scattering indicate that at such excitation field intensities, the relaxation time will be on the order of ~600 fs (see Supplementary Figs 2 and 3 . A detailed discussion of both the numerical simulations for the relaxation rates and the effect of relaxation rates on the HSG spectrum can be found in Supplementary Note 3 ). Hence, we set the relaxation time, ħ /Γ, to 658 fs (Γ=1 meV). The sideband spectrum was calculated for a number of THz field strengths, ranging from 1 kV cm −1 to 4 kV cm −1 . 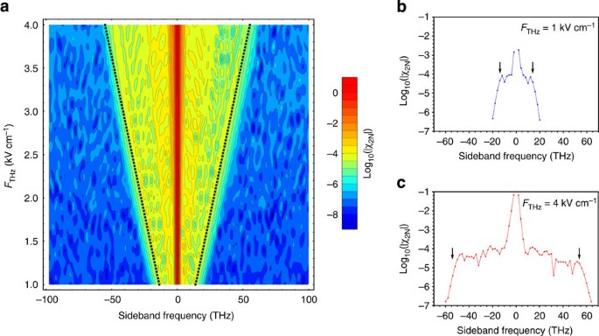Figure 3: Simulated data of the sideband spectrum of a THz-driven bi-layer graphene. (a) Contour plot of the sideband spectrum of THz-driven BLG for different THz field strengths. The colour map gives the logarithm of the normalized sideband amplitude log10(|χ2N|). The dashed black lines give the theoretical sideband cutoffs, ±4Ũp,vc. (b) The sideband spectrum for a THz field of frequency 1 THz and strength of 1 kV cm−1. (c) The sideband spectrum for a THz field of frequency 1 THz and strength 4 kV cm−1. The arrows inbandcmark the location of the theoretical sideband cutoffs, ±4Ũp,vc. Figure 3a shows the sideband spectrum for increasing THz field strength. At a THz field strength of 1 kV cm −1 one can see a plateau, symmetric about the excitation frequency, of width ~28 THz ( Fig. 3b ). As one increases the THz field strength, the plateau grows linearly reaching a width of about 108 THz for a 4 kV cm −1 field ( Fig. 3c ). The amplitude of the sidebands is much smaller than that of the excitation field. In conventional semiconductors, the sideband amplitude has been measured to be about two orders of magnitude smaller than the excitation field [11] . By comparing simulations of HSG in GaAs quantum wells with the experimental data in ref. 11 , we expect that the high sideband amplitudes in BLG to be as much as six orders of magnitude smaller than the excitation field. This comparative reduction in the sideband amplitude compared with conventional semiconductors near the band edge is unsurprising as the process that generates the sidebands in BLG is a quantum process rather than a semi-classical process. Figure 3: Simulated data of the sideband spectrum of a THz-driven bi-layer graphene. ( a ) Contour plot of the sideband spectrum of THz-driven BLG for different THz field strengths. The colour map gives the logarithm of the normalized sideband amplitude log 10 (|χ 2N |). The dashed black lines give the theoretical sideband cutoffs, ±4Ũ p,vc . ( b ) The sideband spectrum for a THz field of frequency 1 THz and strength of 1 kV cm −1 . ( c ) The sideband spectrum for a THz field of frequency 1 THz and strength 4 kV cm −1 . The arrows in b and c mark the location of the theoretical sideband cutoffs, ±4Ũ p,vc . Full size image Plateau cutoff law for linear band materials To further understand the plateau of HSG in BLG, we compare the theoretical model to the equivalent theory for conventional semiconductors. For a parabolic band material, the Schrödinger equation can be solved in a semi-classical approximation to give an expression for the plateau cutoff Δ+3.17 U p (refs 9 , 10 ). One can follow a similar procedure to obtain a cutoff law for BLG (see Supplementary Note 4 ). The E v and E c bands can be expanded to first order about the excitation energy The result is a band structure that resembles a shifted version of monolayer graphene with effective Fermi velocity, . Solving a restricted version of the classical equations of motion for such a system [21] , one obtains a prediction for the plateau cutoffs of 4Ũ p,vc above and below the excitation frequency, with linear ponderomotive energy given by . The dashed black line in Fig. 3a shows the theoretical prediction of the cutoff. One observes good agreement over the full range of THz field strengths simulated. Similarly, the black arrows in Fig. 3b, c mark the theoretical cutoff given by the 4Ũ p,vc cutoff law. Figure 3b shows that at low field strengths the cutoff law is in good agreement with the numerical results. Figure 3c shows that although the cutoff law correctly predicts the high end cutoff, it over-estimates the low end cutoff. The reason for this is that as the bands move towards the Dirac point they deviate from the linear model of equation (1) and, hence, the electron and hole have lower velocities. This leads to the discrepancy observed in Fig. 3c . The advantages of BLG as a material for HSG can be seen by comparison with conventional semiconductors such as GaAs. In order to obtain a bandwidth of about 28 THz with a 1 THz frequency field, one would need a field strength of nearly 14 kV cm −1 (that is, the required THz field intensity for GaAs is ~200 times stronger than for the BLG). Current experiments have used free electron lasers to produce such fields. In principle, such fields can be created in solid-state devices by careful microwave engineering [11] . However, the field reduction offered by BLG will make the engineering of such a device easier as well as resulting in a more compact, lower power design. Another advantage is that BLG has resonant transitions throughout the telecomm frequencies (including all standard band classifications from O-band to U-band, not just the conventional C-band ‘erbium window’), thus allowing broadband modulation at any frequency in this range. This would mean that BLG-based devices could operate optimally over a wide range of frequencies without the need to further tailor the material. Conversely, the GaAs bandgap (which corresponds to a wavelength of ~0.87 μm) is outside the telecomm frequency waveband. Even materials with smaller band gaps (for example, silicon ~1.12 μm, germanium ~1.85 μm) usually need further engineering (either by alloying or via the creation of heterostructures) in order to create a device that is optimally tuned to a particular optical frequency. For exceptionally small band-gap semiconductors (such as InAs ~3.44 μm), a field in the telecomm waveband can also create electron–hole pairs well above the band edge and therefore with high initial velocity. However, the carrier relaxation in such materials, because of the rapid emission of LO phonons (which have energies of tens of meV), would be much faster than in graphene (where the LO phonon energy ~200 meV (ref. 27 )). For optical device applications, one needs to consider the depth of the modulation. Again, the versatile properties of BLG are a bonus and a number of techniques can be employed to increase the amplitude of the sidebands. For example, employing waveguides to increase the interaction length between BLG and the laser, would increase the sideband amplitude and, hence, the modulation depth. Furthermore, owing to the small reflectance of BLG (<0.1%) [15] and the fact that the modulated light is emitted equally in the forward and backward directions, an enhanced modulation depth can be obtain by detection in reflection rather than in transmission. In addition, the compact nature of the process and the fast response time of the effect would both be great advantages of a BLG modulator. The results of this study suggest that biased BLG can provide ultra-broad HSG and, hence, ultrafast modulation of an optical field at THz field strengths low enough for table top sources to be used [28] , [29] , [30] . These results open up the way for ultrafast, HSG-based, optical devices, which, coupled with the remarkable properties of BLG, marks a step towards realizing all optical broadband modulation and optical communication at the Tbit s −1 rate. Time-dependent Schrödinger equation The electron–hole pair wavefunction, , where λ and σ are the spin and valley indices, respectively, was computed using the time-dependent Schrödinger equation with Here, and are the instantaneous valence and conduction band energies, which can be derived using a tight-binding method with nearest neighbour hopping [18] , [19] , [20] . The time-dependent canonical momentum is given by , and and are the interband dipole moment and Berry connection terms [31] , the latter of which is required to preserve gauge invariance. As the driving of the electrons is linear (as opposed to closed orbits) the contribution of the Berry connection term is negligible (see Supplementary Note 5 ). Γ is a phenomenological dephasing rate that accounts for various relaxation mechanisms. For the sake of simplicity, we have not included the Coulomb interaction. This is justified by the condition that the resonant excitation is taken to be far from the band edge and hence off-resonant with the bound state excitations. Furthermore, at such high quasi-momenta, the kinetic term in the Hamiltonian will dominate. Equation (2) was evaluated directly using standard numerical techniques. The resulting polarization is given by with the sideband spectrum calculated via discrete Fourier transform. How to cite this article: Crosse, J. A. et al. Theory of low power ultra-broadband terahertz sideband generation in bi-layer graphene. Nat. Commun. 5:4854 doi: 10.1038/ncomms5854 (2014).